Astrocytic laminin regulates pericyte differentiation and maintains blood brain barrier integrity Blood brain barrier (BBB) breakdown is not only a consequence of but also contributes to many neurological disorders, including stroke and Alzheimer’s disease. How the basement membrane (BM) contributes to the normal functioning of the BBB remains elusive. Here we use conditional knockout mice and an acute adenovirus-mediated knockdown model to show that lack of astrocytic laminin, a brain-specific BM component, induces BBB breakdown. Using functional blocking antibody and RNAi, we further demonstrate that astrocytic laminin, by binding to integrin α2 receptor, prevents pericyte differentiation from the BBB-stabilizing resting stage to the BBB-disrupting contractile stage, and thus maintains the integrity of BBB. Additionally, loss of astrocytic laminin decreases aquaporin-4 (AQP4) and tight junction protein expression. Altogether, we report a critical role for astrocytic laminin in BBB regulation and pericyte differentiation. These results indicate that astrocytic laminin maintains the integrity of BBB through, at least in part, regulation of pericyte differentiation. The blood brain barrier (BBB) is a dynamic network that regulates material exchange between circulatory system and the brain parenchyma, maintaining the homoeostasis of the central nervous system (CNS) [1] . BBB malfunction has been reported in many CNS disorders, including stroke, Alzheimer’s disease, neuroinflammation and various types of infections [2] , [3] , [4] . The BBB is mainly composed of brain microvascular endothelial cells, astrocytic endfeet, pericytes and the basement membrane (BM) [5] . Brain microvascular endothelial cells interconnect via tight junctions, forming the BBB’s primary barrier [6] , [7] . Astrocytes wrap around endothelial cells using their endfeet. Pericytes, sandwiched in endothelial cells and astrocytes, signal to both cell types. Recently, it has been shown that pericytes are necessary for the formation of the BBB during embryogenesis [8] and loss of pericytes leads to compromise of BBB integrity [9] and age-dependent vascular-mediated neurodegeneration in adult mice [10] , suggesting an important role of pericytes in BBB regulation. Although damage to the BM during ischaemic stroke has been linked to BBB breakdown [11] , [12] , the role of the BM, especially that of individual BM components, in the BBB under physiological conditions remains elusive. The BM consists of a mixture of extracellular matrix proteins, including laminin and collagen IV (refs 13 , 14 , 15 , 16 ). Laminin is a trimeric molecule comprising α-, β- and γ-subunits and shows differential expression in the vascular and parenchymal BMs. Brain microvascular endothelial cells generate laminins-411 (α4β1γ1) and -511 (α5β1γ1) [17] , [18] , whereas astrocytes produce laminins-111 (α1β1γ1) and -211 (α2β1γ1) [18] , [19] . These laminin isoforms are all expressed by primary brain capillary pericytes [20] . Since laminins-111 and -211 (astrocytic laminins) are only found in the vasculature of the brain, we hypothesized that astrocytic laminin might be critical for the proper functioning of the BBB. Given the critical regulatory role of astrocytic laminin in vascular smooth muscle cells [21] , we further hypothesize that astrocytic laminin may regulate the differentiation of pericytes, cells that belong to the same lineage as vascular smooth muscle cells. Here we show that lack of astrocytic laminin induces pericyte differentiation from the resting stage to the contractile stage, switching pericyte function from stabilizing the BBB to compromising it. Additionally, lack of astrocytic laminin also abrogates the polarity of astrocytic endfeet and the expression of tight junction proteins in endothelial cells. These results support an important role of astrocytic laminin in the maintenance of BBB integrity. Genetic ablation of glial laminin induces BBB breakdown To investigate the role of astrocytic laminin on BBB integrity, we generated conditional laminin knockout mice (Nγ1-KO) by crossing homozygous floxed laminin γ1 (F/F) mice with Nestin-Cre transgenic mice. Since nestin is expressed by neural progenitor cells, which give rise to neurons and glia, laminin should be deficient in both neurons and glia in the Nγ1-KO mice, which we have validated [21] . To investigate when laminin expression was abrogated, we examined laminin γ1 expression by immunohistochemistry at different stages. At embryonic day 15.5 (E15.5), laminin γ1 level was unaffected in Nγ1-KO brain compared with their littermate controls (Ctr) ( Supplementary Fig. 1 ). At E18.5 and postnatal day 2 (P2), on the other hand, a dramatic decrease of laminin γ1 was observed in Nγ1-KO brain ( Supplementary Fig. 1 ), suggesting that laminin expression was disrupted at late embryonic stages in Nγ1-KO mice. Although brain capillary pericytes have been reported to express nestin [22] , we did not observe nestin and PDGFRβ double-positive cells in the striatum of the Nγ1-KO mice ( Supplementary Fig. 2a ). This nestin antibody specifically labelled neural stem cells in the subgranular zone ( Supplementary Fig. 2b ), suggesting that PDGFRβ-positive pericytes do not express nestin. In addition, EGFP was expressed in brain parenchymal cells (neurons and astrocytes) ( Supplementary Fig. 3b ) but absent in PDGFRβ + pericytes in ROSA26-EGFP +/− Nestin-Cre +/− mice ( Supplementary Fig. 3a ). In Ctr (ROSA26-EGFP +/− Nestin-Cre −/− ) mice, EGFP was totally absent due to the lack of Cre expression ( Supplementary Fig. 3 ). These data suggest that Cre is not expressed in pericytes in the Nγ1-KO mice. To further investigate whether pericytic laminin is affected in this Nγ1-KO mouse line, we isolated primary pericytes from Ctr and mutant brain microvessels and examined their laminin γ1 expression. The purified pericytes were positive for PDGFRβ and CD13 (pericyte markers), while negative for CD31 ( Supplementary Fig. 4a–d ), indicative of high purity. The specificity of the CD31 antibody was validated in purified primary brain capillary endothelial cells ( Supplementary Fig. 4e,f ). Laminin γ 1 mRNA was detected in pericytes from both Ctr and Nγ1-KO mice ( Supplementary Fig. 5a ), and qRT-PCR showed that laminin γ 1 mRNA levels in the pericytes from Nγ1-KO mice was comparable to that from Ctr mice ( Supplementary Fig. 5b ). Consistently, we detected laminin γ1 protein expression in primary pericytes from the Nγ1-KO mice ( Supplementary Fig. 4c and d ), suggesting that pericytic laminin is not affected in the Nγ1-KO mice. We further examined laminin expression in pericytes in vivo using anti-laminin α2 antibody as lack of laminin γ1 leads to intracellular degradation of α and β chains [23] and found that laminin α2 colocalized with CD13 and PDGFRβ in both Ctr and Nγ1-KO mice ( Supplementary Fig. 6 ), although laminin α2 expression level was lower in Nγ1-KO mice. Since laminin α2 is not expressed in endothelial cells, and Nγ1-KO mice [21] and laminin γ1 knockdown mice (see Fig. 4c ) have a deficiency of laminin α2 expression in astrocytes, our results suggest that laminin α2 expression is from pericytes in the Nγ1-KO mice. The lower expression level of laminin α2 in the Nγ1-KO mice is due to the absence of laminin α2 in astrocytes. Altogether, our data suggest that the Nγ1-KO mouse line does not knockout laminin in pericytes. Figure 4: Acute ablation of astrocytic laminin leads to BBB breakdown. Mice were injected with adenovirus as indicated. Seven days after injection, the brains were collected and analysed. 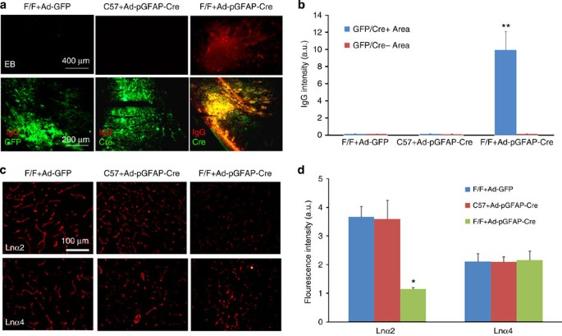Figure 4: Acute ablation of astrocytic laminin leads to BBB breakdown. Mice were injected with adenovirus as indicated. Seven days after injection, the brains were collected and analysed. (a) Evans blue and mouse IgG infiltrate into the brain parenchyma of F/F mice with Ad-pGFAP-Cre injection, but not the Ctr–F/F mice with Ad-GFP injection or C57Bl6 mice with Ad-pGFAP-Cre injection. GFP (for Ad-GFP injected brains) and Cre (for Ad-pGFAP-Cre injected brains) were used to reveal infected regions. (b) Quantification of IgG intensity in GFP/Cre positive and negative areas in adenovirus-injected mouse brains. Data are quantified using nine sections from three animals per group. (c) Laminin is specifically knocked down in astrocytes by adenoviruses. Seven days after adenoviral injection, brains were collected and immunostained for laminin α2 (Lnα2, marker for astrocytic laminin) and α4 (Lnα4, marker for endothelial laminin). Our data show that the adenoviruses we used specifically knocked down astrocytic laminin without affecting endothelial laminin. (d) Quantification of Lnα2 and Lnα4 intensity in the brain parenchyma of the adenovirus-injected mice. Data are quantified using six sections from three animals per group. Scale bars represent 400 μm (EB ina), 200 μm (IgG ina) and 100 μm (c). Data are shown as mean±s.d. *P<0.05 and **P<0.001 versus the Ctr by Student’st-test. ( a ) Evans blue and mouse IgG infiltrate into the brain parenchyma of F/F mice with Ad-pGFAP-Cre injection, but not the Ctr–F/F mice with Ad-GFP injection or C57Bl6 mice with Ad-pGFAP-Cre injection. GFP (for Ad-GFP injected brains) and Cre (for Ad-pGFAP-Cre injected brains) were used to reveal infected regions. ( b ) Quantification of IgG intensity in GFP/Cre positive and negative areas in adenovirus-injected mouse brains. Data are quantified using nine sections from three animals per group. ( c ) Laminin is specifically knocked down in astrocytes by adenoviruses. Seven days after adenoviral injection, brains were collected and immunostained for laminin α2 (Lnα2, marker for astrocytic laminin) and α4 (Lnα4, marker for endothelial laminin). Our data show that the adenoviruses we used specifically knocked down astrocytic laminin without affecting endothelial laminin. ( d ) Quantification of Lnα2 and Lnα4 intensity in the brain parenchyma of the adenovirus-injected mice. Data are quantified using six sections from three animals per group. Scale bars represent 400 μm (EB in a ), 200 μm (IgG in a ) and 100 μm ( c ). Data are shown as mean±s.d. * P <0.05 and ** P <0.001 versus the Ctr by Student’s t -test. Full size image Next, we injected Evans blue intraperitoneally and found leakage of this dye into the brain parenchyma of Nγ1-KO mice but not in Ctr mice ( Fig. 1a ). Consistent with this result, we detected mouse IgG in the brain parenchyma of Nγ1-KO mice but not that of Ctr mice ( Fig. 1b,c ). In a quantitative study, we found more intravenously injected FITC-Dextran (500 kD) in homogenates of Nγ1-KO brains than in those of Ctr brains ( Fig. 1d ). These data indicate that BBB integrity is compromised in Nγ1-KO mice. To determine whether neuronal or glial laminin is responsible for the BBB breakdown phenotype in the Nγ1-KO mice, we also generated conditional neuronal laminin knockout mice, termed Cγ1-KO, by crossing F/F mice with CamKII-Cre transgenic mice. The Cγ1-KO mice showed no signs of BBB disruption [24] ( Fig. 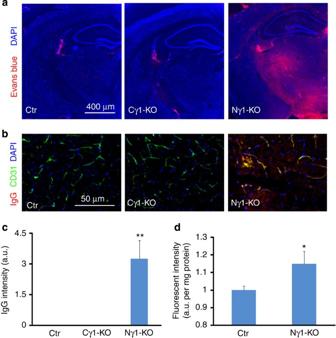1a–c ), suggesting that the BBB breakdown phenotype in the Nγ1-KO mice is due to the lack of laminin in glial cells, not neurons. Figure 1: BBB integrity is compromised in Nγ1-KO mice. Mice were injected with Evans blue intraperitoneally 12 h before the mice were killed. After perfusion, brain sections were used to examine Evans blue directly under fluorescent microscopy and mouse IgG by immunohistochemistry. (a,b) Evans blue (a) and mouse IgG (b) infiltrate the brain parenchyma of Nγ1-KO but not Ctr or Cγ1-KO mice. (c) Quantification of mouse IgG intensity in the brain parenchyma of Nγ1-KO mice. Data are quantified using nine sections from three animals. (d) Quantification of FITC-Dextran in the brain parenchyma. FITC-Dextran (500 kDa) was injected intravenously 12 h before mice were killed. After perfusion, brains were collected and homogenized. Infiltrated FITC-Dextran was quantified using a fluorescence plate reader at 485 nm (n=3). Scale bars represent 400 μm (a) and 50 μm (b). Data are shown as mean±s.d. *P<0.05 and **P<0.001 versus the Ctr by Student’st-test. Figure 1: BBB integrity is compromised in N γ 1-KO mice. Mice were injected with Evans blue intraperitoneally 12 h before the mice were killed. After perfusion, brain sections were used to examine Evans blue directly under fluorescent microscopy and mouse IgG by immunohistochemistry. ( a , b ) Evans blue ( a ) and mouse IgG ( b ) infiltrate the brain parenchyma of Nγ1-KO but not Ctr or Cγ1-KO mice. ( c ) Quantification of mouse IgG intensity in the brain parenchyma of Nγ1-KO mice. Data are quantified using nine sections from three animals. ( d ) Quantification of FITC-Dextran in the brain parenchyma. FITC-Dextran (500 kDa) was injected intravenously 12 h before mice were killed. After perfusion, brains were collected and homogenized. Infiltrated FITC-Dextran was quantified using a fluorescence plate reader at 485 nm ( n =3). Scale bars represent 400 μm ( a ) and 50 μm ( b ). Data are shown as mean±s.d. * P <0.05 and ** P <0.001 versus the Ctr by Student’s t -test. Full size image Changes in individual BBB components in Nγ1-KO mice Astrocytes express AQP4 exclusively at their endfeet to regulate water homoeostasis at the vessel–neuron interface [25] . In Ctr mice, we found high levels of AQP4, which colocalized with endothelial cell marker CD31 in capillaries ( Fig. 2a ), indicating that these astrocytic endfeet were polarized. In Nγ1-KO mice, however, AQP4 expression was dramatically decreased at astrocytic endfeet in capillaries ( Fig. 2a ). Consistently, western blots showed a significant decrease of AQP4 expression in the striatum of Nγ1-KO mice ( Fig. 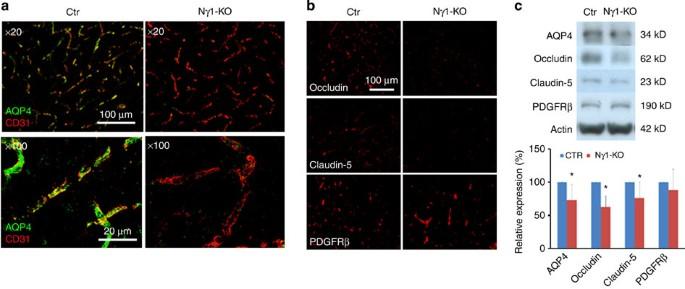2c ), suggesting that the polarity and possibly function of the astrocytic endfeet are lost in Nγ1-KO mouse brains. Figure 2: Individual BBB components are affected in the Nγ1-KO brains. (a) Immunohistochemistry shows that astrocytic endfeet marker AQP4 is expressed at high levels in Ctr mice, but dramatically reduced in Nγ1-KO mice. High-power confocalZprojection images show that AQP4 colocalizes with endothelial cell marker CD31 in Ctr but not Nγ1-KO brains. (b) Occludin and claudin-5, but not PDGFRβ, are significantly decreased in Nγ1-KO brains. (c) Representative western blot of AQP4, occludin, claudin-5, PDGFRβ and actin using striatum lysates from Ctr and Nγ1-KO mice. Full blots of these proteins are shown inSupplementary Fig. 14a. Western blot was quantified by densitometry. All bands were normalized to actin (n=6). Scale bars represent 100 μm (low-magnification images ina,b) and 20 μm (high-magnification images ina). Data are shown as mean±s.d. *P<0.05 versus the Ctr by Student’st-test. Figure 2: Individual BBB components are affected in the N γ 1-KO brains. ( a ) Immunohistochemistry shows that astrocytic endfeet marker AQP4 is expressed at high levels in Ctr mice, but dramatically reduced in Nγ1-KO mice. High-power confocal Z projection images show that AQP4 colocalizes with endothelial cell marker CD31 in Ctr but not Nγ1-KO brains. ( b ) Occludin and claudin-5, but not PDGFRβ, are significantly decreased in Nγ1-KO brains. ( c ) Representative western blot of AQP4, occludin, claudin-5, PDGFRβ and actin using striatum lysates from Ctr and Nγ1-KO mice. Full blots of these proteins are shown in Supplementary Fig. 14a . Western blot was quantified by densitometry. All bands were normalized to actin ( n =6). Scale bars represent 100 μm (low-magnification images in a , b ) and 20 μm (high-magnification images in a ). Data are shown as mean±s.d. * P <0.05 versus the Ctr by Student’s t -test. Full size image Brain microvascular endothelial cells form the primary barrier of the BBB by connecting to each other via tight junctions, where tight junction proteins are expressed [26] , [27] . Although blood vessel density was not affected, as determined by immunostaining for CD31 ( Fig. 2a ), the levels of occludin and claudin-5, two major protein components of tight junctions, were significantly decreased in the capillaries of Nγ1-KO mice ( Fig. 2b ). Consistently, western blots showed diminished expression of occludin and claudin-5 in the striatum of Nγ1-KO mice ( Fig. 2c ), suggesting compromise of the tight junction structure in Nγ1-KO mice. In addition to capillaries, we also examined how loss of astrocytic laminin affected the expression of AQP4 and tight junction proteins in large blood vessels. No decrease of AQP4, occludin and claudin-5 was observed in large vessels in Nγ1-KO mice ( Supplementary Fig. 7 ). Quantitative western blots using large blood vessels showed that claudin-5 was significantly increased in Nγ1-KO mice ( Supplementary Fig. 7 ). These data suggest that loss of astrocytic laminin predominantly affects capillaries in the brain, and defects in capillaries, rather than big blood vessels, are responsible for the BBB leakage phenotype in Nγ1-KO mice. Sandwiched between astrocytes and endothelial cells in capillaries, pericytes also contribute to the integrity of the BBB [8] , [9] , [10] . We examined the expression of PDGFRβ, a pericyte marker, and found no obvious difference between Ctr and Nγ1-KO brains ( Fig. 2b ). Consistent with this result, western blot results did not show a difference in PDGFRβ expression in the striatum of Ctr and Nγ1-KO mice ( Fig. 2c ). To study the ultrastructure of BBB components, we examined brain samples from Ctr and Nγ1-KO mice using electron microscopy (EM). In Ctr mice, pericytes were sandwiched in between well-organized astrocytes and endothelia. The BM between astrocytes and pericytes (blue arrows) and that between pericytes and endothelial cells (green arrowheads) were compact ( Fig. 3a ). In Nγ1-KO mice, however, pericytes changed their morphology ( Fig. 3a ), indicating that pericyte differentiation and/or maturation may be affected. In addition, in Nγ1-KO mice, both BMs were patchy and diffuse (red arrows, Fig. 3a ) and endothelial membrane integrity was compromised (white dots, Fig. 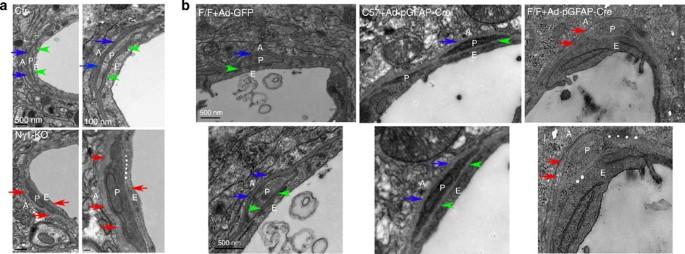3a ), suggesting that glial laminin may regulate pericyte differentiation and maturation. Figure 3: Ultrastructural changes in Nγ1-KO and laminin-knockdown brains. (a) In Ctr mice, the BM between astrocytes and pericytes (blue arrows) and that between pericytes and endothelial cells (green arrowheads) are compact and pericytes are tightly attached to endothelial cells. In the Nγ1-KO mice, however, pericytes change their morphology and both BMs show a patchy and diffused pattern (red arrows). Moreover, the endothelial membrane integrity is compromised at some places (white dots) in Nγ1-KO mice. (b) In Ctr mice (F/F+Ad-GFP and C57+Ad-pGFAP-Cre), pericytes are surrounded by nicely aligned and compact BMs secreted by both astrocytes (blue arrows) and endothelial cells (green arrowheads). In astrocytic laminin-knockdown mice (F/F+Ad-pGFAP-Cre), on the other hand, pericytes change their morphology and both BMs become patchy and diffuse (red arrows). In addition, the BMs are hard to define at some places and the membrane integrity is severely compromised in these astrocytic laminin-knockdown mice (white dots). A, astrocytes; P, pericytes; E, endothelia. Scale bars represent 500 nm (low-magnification images inaon the left andb), and 100 nm (high-magnification images inaon the right). Figure 3: Ultrastructural changes in N γ 1-KO and laminin-knockdown brains. ( a ) In Ctr mice, the BM between astrocytes and pericytes (blue arrows) and that between pericytes and endothelial cells (green arrowheads) are compact and pericytes are tightly attached to endothelial cells. In the Nγ1-KO mice, however, pericytes change their morphology and both BMs show a patchy and diffused pattern (red arrows). Moreover, the endothelial membrane integrity is compromised at some places (white dots) in Nγ1-KO mice. ( b ) In Ctr mice (F/F+Ad-GFP and C57+Ad-pGFAP-Cre), pericytes are surrounded by nicely aligned and compact BMs secreted by both astrocytes (blue arrows) and endothelial cells (green arrowheads). In astrocytic laminin-knockdown mice (F/F+Ad-pGFAP-Cre), on the other hand, pericytes change their morphology and both BMs become patchy and diffuse (red arrows). In addition, the BMs are hard to define at some places and the membrane integrity is severely compromised in these astrocytic laminin-knockdown mice (white dots). A, astrocytes; P, pericytes; E, endothelia. Scale bars represent 500 nm (low-magnification images in a on the left and b ), and 100 nm (high-magnification images in a on the right). Full size image Lack of astrocytic laminin leads to BBB breakdown Glia includes astrocytes and oligodendrocytes. Astrocytic endfeet wrap around endothelial cells and pericytes, while oligodendrocytes do not participate in the formation of BBB directly. Therefore, we hypothesized that it is the lack of astrocytic laminin that induces BBB disruption. To test this hypothesis, we acutely knocked down the expression of laminin specifically in astrocytes by injecting adenovirus expressing Cre under a GFAP promoter (Ad-pGFAP-Cre, kindly provided by Dr Alvarez-Buylla) into adult F/F mice. Wild-type (C57Bl6) mice injected with Ad-pGFAP-Cre and F/F mice injected with adenovirus expressing GFP only (Ad-GFP) were used as Ctr. To examine the cell types expressing Cre after Ad-pGFAP-Cre injection, we performed immunohistochemistry on brains collected 7 days after injection. We found that Cre colocalized with the astrocyte marker GFAP, but not the neuronal marker TUJ1 or pericyte marker PDGFRβ ( Supplementary Fig. 8 ), indicating Cre is specifically expressed in astrocytes after injection. Leakage of Evans blue and mouse IgG was observed in F/F mice 7 days after Ad-pGFAP-Cre injection, but not in Ctr ( Fig. 4a ). We further noticed that extravasated IgG colocalized well with Cre in F/F mice injected with Ad-pGFAP-Cre ( Fig. 4a ). The quantification of IgG intensity showed a significant increase in Cre positive area in F/F mice injected with Ad-pGFAP-Cre, but not the Ctr ( Fig. 4b ). GFP (for F/F+Ad-GFP) and Cre (for C57+Ad-pGFAP-Cre and F/F+Ad-pGFAP-Cre) immunohistochemistry revealed similar size of infected areas ( Fig. 4a ), suggesting that BBB breakdown in Ad-pGFAP-Cre injected F/F mice was not due to different virus titre/dose. These data suggest that acute ablation of astrocytic laminin alone is sufficient to induce BBB breakdown. To validate that the disruption of BBB integrity was actually due to the lack of astrocytic laminin, we examined the expression of laminin in these mice. Given the differential expression of laminin isoforms in the neurovascular unit, laminin α2 and α4 were used as markers for astrocytic and endothelial laminin, respectively. Wild-type mice with Ad-pGFAP-Cre injection and F/F mice with Ad-GFP injection did not show any changes in the expression of laminins α2 and α4 ( Fig. 4c,d ). Injection of Ad-pGFAP-Cre into F/F mice, however, decreased the expression of laminin α2 without affecting laminin α4 expression ( Fig. 4c,d ), indicating specific knockdown of laminin in astrocytes. In addition, we also examined TUNEL staining 7, 30 and 60 days after adenovirus injection. No TUNEL-+ cells were found at the injection site ( Supplementary Fig. 9 ), whereas recombinant DNase I pretreated brain sections showed a large number of TUNEL + cells (positive Ctr). These results suggest that the conditions we used did not cause apoptotic cell death, and that astrocytic laminin is necessary for the maintenance of BBB integrity. Lack of astrocytic laminin affects BBB components We next investigated how lack of astrocytic laminin affects individual components of the BBB. Like Nγ1-KO mice, APQ4 expression was dramatically decreased in F/F mice injected with Ad-pGFAP-Cre, but not in the Ctr ( Fig. 5a ). The expression levels of occludin ( Fig. 5b ) and claudin-5 ( Fig. 5c ) followed the same trend. 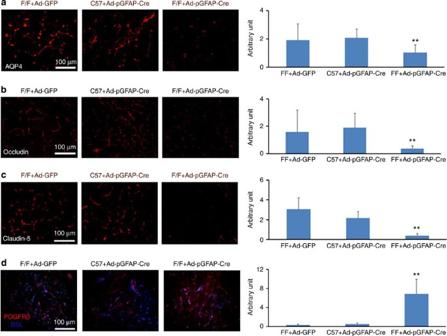Figure 5: Acute ablation of astrocytic laminin affects individual BBB components. Mice were injected with adenovirus as indicated. Seven days after injection, the brains were collected and analysed. (a) Immunohistochemistry shows that astrocytic endfeet marker AQP4 is significantly decreased in F/F mice with Ad-pGFAP-Cre injection, but not in the Ctr–F/F mice with Ad-GFP injection or C57 mice with Ad-pGFAP-Cre injection. AQP4 fluorescence intensity was quantified using 12–13 random sections from three or more mice per group. (b,c) Immunohistochemistry shows that occludin (b) and claudin-5 (c) are significantly decreased in F/F mice with Ad-pGFAP-Cre injection, but not in the Ctr. The fluorescence intensity of these proteins was quantified using 9–13 random sections from at least three mice per group. (d) Immunohistochemistry shows that the pericyte marker PDGFRβ is significantly increased in F/F mice with Ad-pGFAP-Cre injection, but not in the Ctr. PDGFRβ fluorescence intensity was quantified using 11–12 random sections from at least three mice per group. Scale bars represent 100 μm. Data are shown as mean±s.d. **P<0.001 versus the Ctr by Student’st-test. Figure 5: Acute ablation of astrocytic laminin affects individual BBB components. Mice were injected with adenovirus as indicated. Seven days after injection, the brains were collected and analysed. ( a ) Immunohistochemistry shows that astrocytic endfeet marker AQP4 is significantly decreased in F/F mice with Ad-pGFAP-Cre injection, but not in the Ctr–F/F mice with Ad-GFP injection or C57 mice with Ad-pGFAP-Cre injection. AQP4 fluorescence intensity was quantified using 12–13 random sections from three or more mice per group. ( b , c ) Immunohistochemistry shows that occludin ( b ) and claudin-5 ( c ) are significantly decreased in F/F mice with Ad-pGFAP-Cre injection, but not in the Ctr. The fluorescence intensity of these proteins was quantified using 9–13 random sections from at least three mice per group. ( d ) Immunohistochemistry shows that the pericyte marker PDGFRβ is significantly increased in F/F mice with Ad-pGFAP-Cre injection, but not in the Ctr. PDGFRβ fluorescence intensity was quantified using 11–12 random sections from at least three mice per group. Scale bars represent 100 μm. Data are shown as mean±s.d. ** P <0.001 versus the Ctr by Student’s t -test. Full size image Interestingly, F/F mice with Ad-pGFAP-Cre injection showed upregulation of PDGFRβ compared with the Ctr ( Fig. 5d ), suggesting that astrocytic laminin may affect the proliferation or differentiation of pericytes. To investigate this further, we examined the expression of Ki67, a proliferation marker. Neither total Ki67 + nor Ki67 + PDGFRβ + cell numbers in Ad-pGFAP-Cre injected F/F mice showed a difference compared with the Ctr ( Supplementary Fig. 10 ), suggesting that differentiation, rather than proliferation, is responsible for the enhanced expression of PDGFRβ in the acute astrocytic laminin knockdown model. We also performed EM analysis using brain samples from these adenovirus-injected mice ( Fig. 3b ). In the Ctr, astrocytes, pericytes and endothelial cells were well-organized. Pericytes were surrounded by BMs secreted by endothelial cells (green arrowheads) and astrocytes (blue arrows) ( Fig. 3b ). In astrocytic laminin-knockdown mice (F/F+Ad-pGFAP-Cre), however, morphological change was observed in capillary pericytes ( Fig. 3b ). Similar to Nγ1-KO mice, these astrocytic laminin-knockdown mice showed patchy and diffuse BMs (red arrows, Fig. 3b ) and the BMs were difficult to define at some places ( Fig. 3b ). Additionally, pericyte and endothelial membrane integrity was disrupted and unclear at certain locations in these mice (white dots, Fig. 3b ). Altogether, our data suggest that astrocytic laminin regulates pericyte differentiation and maturation. Laminin-111 blockage promotes pericyte differentiation Pericytes are multipotent stem and/or progenitor cells, which can be differentiated into many different cells types in vitro [28] , [29] . Although markers for pericytes at different differentiation stages are not well defined, smooth muscle actin-α (SMA) is used as a marker of differentiation [30] and SMA high pericytes are more often found in abnormal conditions [28] , including fibrotic tissue and tumours. It has been shown that only a small portion of pericytes are positive for SMA in the brain in vivo [29] , [31] . In primary cultures, <5% of freshly isolated brain capillary pericytes express SMA [14] , [32] , but all of them become SMA+ by day 7 (refs 33 , 34 , 35 ). These results suggest that components from the brain, such as the astrocytic BM, a brain-specific protein mixture that has direct contact with pericytes, may regulate the expression of SMA in pericytes [36] and hence pericyte differentiation. Together with our EM results and in vivo data, we further hypothesized that astrocytic laminin inhibits SMA expression in pericytes, thereby preventing pericyte differentiation. To test this hypothesis, we plated primary pericytes on laminin-111 (astrocytic laminin)-coated plates and treated them with laminin-111 blocking antibody or Ctr IgG. Consistent with our in vivo data, laminin-111 blockage induced an upregulation of PDGFRβ ( Fig. 6a ). SMA and another contractile protein SM22-alpha (SM22-α) were also increased after laminin-111 blockage ( Fig. 6a ), suggesting that laminin-111 maintains pericytes in an undifferentiated or less differentiated stage with low levels of contractile proteins. 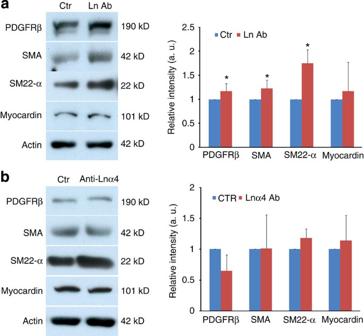Figure 6: Laminin-111 but not laminin-α4 blocking antibody affects pericyte differentiation. (a) Immunoblots show that laminin-111 blockage (Ln Ab) significantly enhances the expression of PDGFRβ, SMA and SM22-α, but not myocardin in pericytes. Full blots of these proteins are shown inSupplementary Fig. 14b. Rabbit IgG treated cells were used as a Ctr. All bands were normalized to actin (n=5–6). (b) Immunoblots show that laminin-α4 blockage (anti-Lnα4) does not change the expression of PDGFRβ, SMA, SM22-α or myocardin in pericytes. Full blots of these proteins are shown inSupplementary Fig. 14c. Rabbit IgG-treated cells were used as a Ctr. All bands were normalized to actin (n=3). Data are shown as mean±s.d. *P<0.05 versus the Ctr by Student’st-test. Figure 6: Laminin-111 but not laminin-α4 blocking antibody affects pericyte differentiation. ( a ) Immunoblots show that laminin-111 blockage (Ln Ab) significantly enhances the expression of PDGFRβ, SMA and SM22-α, but not myocardin in pericytes. Full blots of these proteins are shown in Supplementary Fig. 14b . Rabbit IgG treated cells were used as a Ctr. All bands were normalized to actin ( n =5–6). ( b ) Immunoblots show that laminin-α4 blockage (anti-Lnα4) does not change the expression of PDGFRβ, SMA, SM22-α or myocardin in pericytes. Full blots of these proteins are shown in Supplementary Fig. 14c . Rabbit IgG-treated cells were used as a Ctr. All bands were normalized to actin ( n =3). Data are shown as mean±s.d. * P <0.05 versus the Ctr by Student’s t -test. Full size image Although pericytes and vascular smooth muscle cells belong to the same lineage and category [28] , they respond differently to laminin. It has been shown that laminin promotes the expression of contractile proteins in vascular smooth muscle cells [37] , [38] and this effect is mediated by transcriptional factor myocardin [39] , [40] . To investigate whether the same signalling pathway is activated in pericytes, we examined myocardin levels in pericytes after laminin-111 blocking antibody treatment. Myocardin level was not affected by laminin-111 blockage ( Fig. 6a ), suggesting that pericytes and vascular smooth muscle cells use different mechanisms to regulate contractile protein expression. Additionally, pericytes were treated with conditioned medium from astrocytes, and the expression of PDGFRβ, SMA, SM22-α and myocardin was examined by western blot. As expected, none of these markers was affected ( Supplementary Fig. 11 ), suggesting that the increased expression of PDGFRβ and contractile proteins is not due to soluble factors secreted by astrocytes. To exclude the possibility that pericyte-secreted laminin-411 also contributes to the enhanced expression of PDGFRβ and contractile proteins, we applied laminin α4-specific blocking antibody to cultures. Blockage of laminin α4 did not affect any of the proteins examined ( Fig. 6b ), suggesting that it is astrocytic laminin that regulates the differentiation of pericytes. Laminin regulates pericyte differentiation via integrin α2 To indentify the receptor(s) that mediates astrocytic laminin-induced pericyte differentiation, we treated primary pericytes plated in laminin-111 coated plates with functional blocking antibodies to integrin α2 (ITGA2) and integrin β1 (ITGB1). ITGA2 blockage significantly enhanced the expression of PDGFRβ, SMA and SM-22α, while ITGB1 blockage did not affect the expression of these markers ( Fig. 7a ), suggesting that ITGA2 but not ITGB1 is involved in astrocytic laminin-induced pericyte differentiation. The expression of myocardin, as expected, was not affected by these blocking antibodies ( Fig. 7a ), again suggesting that pericytes and vascular smooth muscle cells have different regulatory machinery in contractile protein expression. 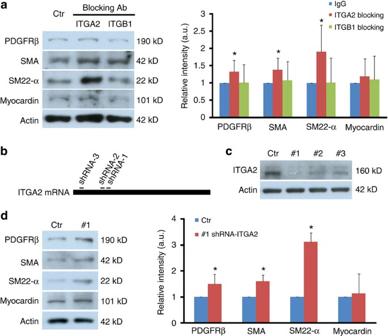Figure 7: Astrocytic laminin mediates pericyte differentiation via integrin α2. (a) Immunoblots show that integrin α2 blockage (ITGA2) but not integrin β1 blockage significantly increases the expression of PDGFRβ, SMA and SM22-α, but not myocardin in pericytes. Full blots of these proteins are shown inSupplementary Fig. 14d. Rabbit IgG-treated cells were used as a Ctr. All bands were normalized to actin (n=6). (b) Schematic diagram of shRNA designed to target ITGA2 mRNA. (c) Immunoblot analysis shows that all three ITGA2-specific shRNAs (#1–3) dramatically reduce ITGA2 at protein level and ITGA2-specific shRNA-3 (#1) is the most efficient one. Full blots of ITGA2 and actin are shown inSupplementary Fig. 14e. Scramble shRNA was used as a Ctr. (d) Immunoblot analysis shows that transduction of pericytes with lenti-shRNA-1 (#1) significantly enhances the expression of PDGFRβ, SMA and SM22-α, but does not affect myocardin level. Full blots of these proteins are shown inSupplementary Fig. 14f. Scramble shRNA was used as a Ctr. All bands were normalized to actin (n=4–5). Data are shown as mean±s.d. *P<0.05 versus the Ctr by Student’st-test. Figure 7: Astrocytic laminin mediates pericyte differentiation via integrin α2. ( a ) Immunoblots show that integrin α2 blockage (ITGA2) but not integrin β1 blockage significantly increases the expression of PDGFRβ, SMA and SM22-α, but not myocardin in pericytes. Full blots of these proteins are shown in Supplementary Fig. 14d . Rabbit IgG-treated cells were used as a Ctr. All bands were normalized to actin ( n =6). ( b ) Schematic diagram of shRNA designed to target ITGA2 mRNA. ( c ) Immunoblot analysis shows that all three ITGA2-specific shRNAs (#1–3) dramatically reduce ITGA2 at protein level and ITGA2-specific shRNA-3 (#1) is the most efficient one. Full blots of ITGA2 and actin are shown in Supplementary Fig. 14e . Scramble shRNA was used as a Ctr. ( d ) Immunoblot analysis shows that transduction of pericytes with lenti-shRNA-1 (#1) significantly enhances the expression of PDGFRβ, SMA and SM22-α, but does not affect myocardin level. Full blots of these proteins are shown in Supplementary Fig. 14f . Scramble shRNA was used as a Ctr. All bands were normalized to actin ( n =4–5). Data are shown as mean±s.d. * P <0.05 versus the Ctr by Student’s t -test. Full size image To confirm the role of ITGA2 in pericyte differentiation, we genetically ablated ITGA2 expression using a shRNA-mediated knockdown technique. Three shRNA sequences targeting ITGA2 (Lenti-shRNA-1-3) and one scramble sequence (Lenti-shRNA-scramble; Ctr) were used ( Fig. 7b ). Seven days after transduction, we detected a significant decrease of ITGA2 expression by western blot, where Lenti-shRNA-3 (#1) was the most efficient ( Fig. 7c ). Next, we transduced pericytes with #1 and Lenti-shRNA-scramble for 7 days and found that #1 significantly increased the expression of PDGFRβ, SMA and SM-22α, without affecting myocardin level ( Fig. 7d ). These data suggest that ITGA2 is indeed the receptor that mediates astrocytic laminin-induced pericyte differentiation and myocardin does not regulate contractile protein expression in pericytes. Astrocytic laminin regulates pericyte differentiation in vivo To investigate whether astrocytic laminin regulates pericyte differentiation in vivo , we first examined SMA expression in PDGFRβ-positive pericytes in Ctr and Nγ1-KO mice. In Ctr brains, no SMA expression was found in PDGFRβ-positive pericytes ( Fig. 8a ). In Nγ1-KO mice, however, SMA and PDGFRβ double-positive pericytes were observed in the deep brain regions, such as striatum, basal ganglia, thalamus and hypothalamus, but not in the cortex or hippocampus ( Fig. 8a ). The quantification of SMA intensity normalized by PDGFRβ intensity revealed a significant difference between Ctr and Nγ1-KO mice in the deep brain regions, but not in cortex or hippocampus ( Fig. 8a ). Next, we examined SMA expression in capillary pericytes in the acute model. GFP and Cre immunohistochemistry were used to locate the infection site. Ad-pGFAP-Cre injection in F/F mice induced SMA expression in PDGFRβ-positive capillary pericytes, whereas pericytes from Ctr animals were SMA-negative ( Fig. 8b ). Quantification showed a significant increase of SMA expression in capillary pericytes in Cre-positive region ( Fig. 8b ). Altogether, our data suggest that lack of astrocytic laminin induces differentiation of capillary pericytes in vivo . 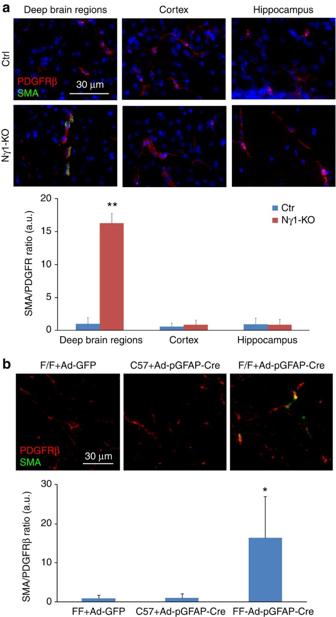Figure 8: Loss of astrocytic laminin increases the expression of SMA by capillary pericytesin vivo. Immunohistochemistry analysis shows significant enhanced SMA expression in PDGFRβ-positive capillary pericytes in deep brain regions of Nγ1-KO mice (a). In the Ctr brain or the cortex and hippocampus of Nγ1-KO mice, however, no SMA-positive capillary pericytes are observed (a). In addition, acute ablation of astrocytic laminin by intracranial injection of adenoviruses significantly elevates the expression of SMA in PDGFRβ-positive pericytes (b). The quantification was performed by calculating the ratio of SMA intensity to PDGFRβ intensity in 9–10 random sections from at least three mice per group. Scale bars represent 30 μm. Data are shown as mean±s.d. *P<0.05 and **P<0.01 versus Ctr by Student’st-test. Figure 8: Loss of astrocytic laminin increases the expression of SMA by capillary pericytes in vivo . Immunohistochemistry analysis shows significant enhanced SMA expression in PDGFRβ-positive capillary pericytes in deep brain regions of Nγ1-KO mice ( a ). In the Ctr brain or the cortex and hippocampus of Nγ1-KO mice, however, no SMA-positive capillary pericytes are observed ( a ). In addition, acute ablation of astrocytic laminin by intracranial injection of adenoviruses significantly elevates the expression of SMA in PDGFRβ-positive pericytes ( b ). The quantification was performed by calculating the ratio of SMA intensity to PDGFRβ intensity in 9–10 random sections from at least three mice per group. Scale bars represent 30 μm. Data are shown as mean±s.d. * P <0.05 and ** P <0.01 versus Ctr by Student’s t -test. Full size image The phenotypes observed in Nγ1-KO mice are brain-specific To investigate whether the capillary leakage and pericyte differentiation phenotypes in Nγ1-KO mice are unique to the brain, we also performed permeability and pericyte differentiation assays in peripheral organs, including liver, kidney and spleen. The levels of IgG in liver, kidney, and spleen were similar between Ctr and Nγ1-KO mice ( Supplementary Fig. 12a ), suggesting that capillary permeability was not affected in the peripheral system in Nγ1-KO mice. Next, we further examined SMA expression in PDGFRβ-positive pericytes and found no difference between Ctr and Nγ1-KO mice in these organs ( Supplementary Fig. 12b ), suggesting that pericyte differentiation was not modified in the peripheral system in Nγ1-KO mice. Altogether, our data indicate that the phenotypes we observed in Nγ1-KO mice are brain-specific, probably due to the exclusive distribution of astrocytes in the brain. In as early as 1963, researchers noticed that emigrating leukocytes are more often found between the endothelium and BM than in the progress of passing between endothelial cells [41] , suggesting that the BM acts as a distinct barrier of the BBB and offers resistance to migrating leukocytes [41] , [42] . However, the normal physiological roles of the BM and its components in BBB regulation remain elusive, probably due to the complexity of BM composition and the lack of animal models and research tools. Using conditional laminin γ1 knockout mice and an adenovirus-mediated astrocyte-specific laminin knockdown technique, we report that lack of astrocytic laminin leads to breakdown of the BBB. Further mechanistic studies showed that lack of astrocytic laminin affected astrocytic endfeet polarity, pericyte differentiation and endothelial tight junction protein expression. This is, to our knowledge, the first study reporting a crucial role of astrocytic laminin on the maintenance of BBB integrity in physiological condition. Our studies also for the first time, to our knowledge, reveal that laminin-111 actively regulates the differentiation of pericytes. Our data show that BBB breakdown and pericyte differentiation are predominantly found in deep brain regions, including striatum, basal ganglia, thalamus and hypothalamus, and rarely found in cortex and hippocampus in the Nγ1-KO mice. The exact mechanism responsible for this regional difference is not clear. However, pia matter may be one possible explanation. Pia matter synthesizes laminin-111 and 211 (astrocytic laminin) and covers blood vessels in surface regions, including cortex [43] , [44] . In the surface brain regions of Nγ1-KO mice, the loss of astrocytic laminin could be compensated by laminin from pia matter. In deep brain regions, however, this compensation mechanism does not exist due to the lack of pia matter, leading to BBB breakdown and pericyte differentiation. Another possibility is that the astrocyte heterogeneity may contribute to the regional difference. Astrocytes from different brain regions have different morphology, gene expression profiles and biological functions [45] , [46] . It is possible that the unique properties of astrocytes in deep brain regions (anatomical structure, gene expression profiles, relationship to pericytes and function) are responsible for the regional difference. Astrocytes, the most abundant cell type in the brain, wrap around endothelial cells and pericytes with their polarized endfeet, participating in the formation of the BBB. AQP4, a water channel protein exclusively expressed on astrocytic endfeet to regulate water homoeostasis at the vessel–neuron interface [25] , has been shown to play an important role in BBB regulation [9] , [47] , [48] . Mice deficient in pericytes lack an astrocytic BM, have a leaky BBB and lose AQP4 expression in astrocytic endfeet [9] . BBB compromise has also been reported in the dystrophin-deficient mdx mice, which have age-dependent reduction of AQP4 expression in astrocytes [47] , [48] . In addition, patchy distribution of AQP4 and other astrocyte endfeet proteins is also reported in mice lacking astrocytic integrin β1, a major receptor for astrocytic laminin [49] . Consistent with these reports, we found decrease of AQP4 and BBB breakdown in mice lacking astrocytic laminin, indicating a pivotal role of astrocytic laminin in the regulation of astrocytic polarity and BBB function. Recently, pericytes have been shown to play an important role in the regulation of vascular permeability [9] , [10] and formation of the BBB [8] . Acute ablation of laminin expression by adenoviral injection compromised BBB integrity, upregulated expression of the pericyte marker PDGFRβ, but did not affect pericyte proliferation, linking laminin to pericyte differentiation. Although many cellular markers, including SMA, PDGFRβ and CD13 have been suggested for pericytes [28] , [50] , the expression of these markers is highly dynamic depending on the developmental stage and pathological conditions [28] . Additionally, other cells also share these markers with pericytes [28] . We showed in vitro that blockage of laminin-111 converted pericytes from a stage with low levels of SMA, SM22-α and PDGFRβ, to one with high levels of these proteins, suggesting that pericytes have at least two differentiation stages (contractile protein low and high ) and that laminin-111 inhibits their differentiation to the contractile protein high stage. Furthermore, we observed that SMA was expressed in capillary pericytes in deep brain regions of Nγ1-KO and Ad-pGFAP-Cre injected F/F mice but not Ctr brains, suggesting that astrocytic laminin is inhibitory to pericyte differentiation in vivo and that the differentiated SMA high pericytes destabilize BBB integrity. These results are consistent with the report that TGFβ-treated pericytes, which express high levels of SMA, decreased BBB integrity, whereas bFGF-treated pericytes, which express low levels of SMA, stabilize the barrier integrity [30] . Goritz et al. [51] classified pericytes into two subclasses: type A (SMA − , Glast + , Desmin − and PDGFRβ + ) and type B (SMA + , Glast − , Desmin + and PDGFRβ + ). They reported that SMA − type A pericytes left blood vessel wall and became SMA + in a spinal cord injury model [51] , again suggesting that SMA + pericytes destabilize BBB integrity. Taken together, we propose a model showing how astrocytic laminin affects pericyte differentiation and BBB integrity ( Fig. 9 ). Pericytes embedded in BMs express low levels of PDGFRβ and contractile proteins (SMA and SM22-α), defined as resting stage. Upon injuries that cause loss of BM, especially laminin-111, pericytes change their morphology and switch to a stage with high levels of contractile proteins and PDGFRβ, defined as the contractile stage. The differentiation from the resting stage to the contractile stage changes the functions of pericytes from barrier stabilization to barrier disruption. Furthermore, our data suggest that this functional conversion is mediated by ITGA2. 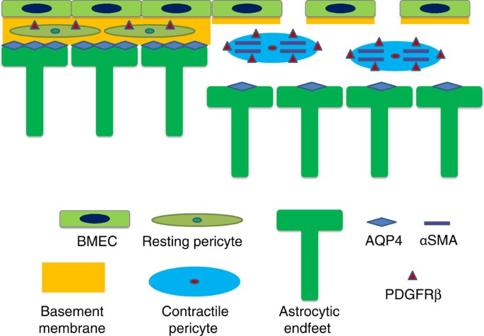Figure 9: Proposed model of how astrocytic laminin affects pericyte differentiation and BBB integrity. Under physiological conditions, pericytes are surrounded in the BMs produced by both astrocytes and endothelial cells. They are in the resting stage, signified by the low expression levels of PDGFRβ and contractile proteins (SMA and SM-22α). When astrocytic laminin is lost during pathological conditions, pericytes hypertrophy and the expression levels of PDGFRβ and contractile proteins are enhanced, switching pericytes to their contractile stage. This process is mediated by integrin α2. This transition changes the function of pericytes from BBB stabilization to BBB disruption. In addition, lack of astrocytic laminin also leads to reduction of AQP4 expression at astrocytic endfeet. Together these effects result in decreased expression of tight junction proteins on endothelial cells, leading to BBB breakdown and subsequent damage. Figure 9: Proposed model of how astrocytic laminin affects pericyte differentiation and BBB integrity. Under physiological conditions, pericytes are surrounded in the BMs produced by both astrocytes and endothelial cells. They are in the resting stage, signified by the low expression levels of PDGFRβ and contractile proteins (SMA and SM-22α). When astrocytic laminin is lost during pathological conditions, pericytes hypertrophy and the expression levels of PDGFRβ and contractile proteins are enhanced, switching pericytes to their contractile stage. This process is mediated by integrin α2. This transition changes the function of pericytes from BBB stabilization to BBB disruption. In addition, lack of astrocytic laminin also leads to reduction of AQP4 expression at astrocytic endfeet. Together these effects result in decreased expression of tight junction proteins on endothelial cells, leading to BBB breakdown and subsequent damage. Full size image Unlike pericytes, which cover capillaries [28] , vascular smooth muscle cells are found in arteries and arterioles. Vascular smooth muscle cells can switch between two phenotypes: a synthetic phenotype and a contractile phenotype [52] . We and others [21] , [37] , [38] have shown that laminin induces SMA expression in vascular smooth muscle cells, promoting a contractile phenotype. Altogether, these data suggest a different role of laminin on pericytes and vascular smooth muscle cells—laminin promotes the differentiation of vascular smooth muscle cells to the contractile phenotype, but maintains pericytes in their resting stage. These results can be explained given the location and function of these cells. Vascular smooth muscle cells regulate arterial blood pressure and local blood flow [52] . Thus, the contractile phenotype should be maintained under physiological conditions. Pericytes actively regulate BBB integrity [8] , [9] , [10] , [28] , although they may also constrict capillaries under pathological conditions [53] , [54] , [55] . Given that the size of a capillary is <8 μm [56] , which allows the passage of only one red blood cell at a time, it is logical for pericytes to have a resting state under physiological conditions to allow patency of the vessel. The next question then becomes: how does laminin exert different roles in pericytes and vascular smooth muscle cells? Our data show that ITGA2 actively regulates pericyte differentiation, but it is not expressed in vascular smooth muscle cells ( Supplementary Fig. 13 ). Additionally, myocardin, a transcriptional factor known to regulate vascular smooth muscle differentiation, is not affected by laminin-111 blockage or ITGA2 blockage/knockdown in pericytes, suggesting that pericytes and vascular smooth muscle cells use different molecular mechanisms to regulate their differentiation. Our results showed that PDGFRβ levels were dramatically increased in the adenoviral injection experiments, but not affected in Nγ1-KO brains. This discrepancy could be due to compensatory mechanisms. Adenoviral injection in adult mice knocks down the expression of laminin γ1 acutely, while long-term loss of laminin γ1 is found in the Nγ1-KO mice. The long-term loss of laminin γ1 may activate compensatory mechanisms, which act to decrease PDGFRβ levels. In the acute model, on the contrary, these mechanisms may not yet be activated. Similar compensation was reported previously [57] , [58] , [59] . No abnormalities of neural stem cell behaviour were reported in integrin α6 −/− mice [59] or mice lacking ITGB1 specifically in these cells [58] . Transient ablation of ITGB1 in embryonic brains by blocking antibody, however, resulted in abnormal neural stem cell proliferation, dystrophic radial glia fibres and substantial layering defects in the postnatal neocortex [57] . In summary, we report a critical role of astrocytic laminin in the maintenance of BBB integrity under normal conditions. Astrocytic laminin polarizes astrocytic endfeet, inhibits pericyte differentiation and induces/maintains tight junction protein expression in endothelial cells. Our data provide novel molecular targets to manipulate BBB integrity and thus promote the development of effective drugs or therapeutic reagents for many CNS diseases. Animals Wild-type (C57BL/6), homozygous floxed laminin γ1 (F/F) mice, Nestin-Cre, CaMKII-Cre, GFAP-Cre and ROSA26-EGFP transgenic mice were maintained in the Comparative Biosciences Center at The Rockefeller University with free access to water and food. F/F mice were crossed with these transgenic mouse lines to generate conditional laminin knockout mice (laminin expression was not successfully decreased in astrocytes in F/F GFAP-Cre mice). Two to four-month-old knockout mice (both genders) and age-matched Ctr (both genders) were used to perform experiments. Experimental procedures were in accordance with the NIH guide for care and use of animals and approved by the Animal Care and Use Committee at The Rockefeller University. Cell culture and treatments Primary human brain vascular pericytes, vascular smooth muscle cells and astrocytes were purchased from ScienCell and maintained in their respective media (ScienCell) and/or DMEM supplemented with 10% FBS. When cells reached 70% confluence, dialyzed anti-laminin-111 blocking antibody (Sigma, L9393, 25 μg ml −1 ), anti-laminin α4 blocking antibody 2A3 (kindly provided by Dr Jonathan Jones, non-diluted), anti-ITGA2 blocking antibody (Millipore, MAB1950Z, 25 μg ml −1 ), anti-ITGB1 blocking antibody (BD, 555002, 25 μg ml −1 ) or anti-rabbit IgG (Sigma, R5506, 25 μg ml −1 ) were added to the media. Media was replaced every 2 days. On day 7, cells were collected and lysed with RIPA buffer (50 mM Tris, pH 7.4, 1% NP-40, 0.5% Na-deoxycholate, 1% SDS, 150 mM NaCl, 2 mM EDTA, 1 × protease inhibitor cocktail and 1 × phosphatase inhibitor cocktail). Primary brain pericytes were isolated and cultured as described [22] , [60] . Briefly, brains from 2–4 month-old Ctr and Nγ1-KO mice (both males and females) were collected under aseptic conditions, followed by homogenization in DMEM+5% FBS. After centrifugation, the pellet was resuspended in 17% dextran solution and centrifuged at 6,000 g for 15 min at 4 °C. Blood vessels were collected at the bottom and resuspended in DMEM+5% FBS. These vessels were sequentially filtered through 100-μm and 40-μm cell strainers. Microvessels trapped by 40-μm cell strainer were collected and digested with 1 mg ml −1 collagenase/dispase (Roche) for 4 h at 37 °C. After digestion, the vessels were triturated with pipette and plated in uncoated plastic plates. After 8 h, unattached cells were removed by shaking and gentle pipetting. The attached pericytes were then grown in pericyte medium (ScienCell). Large blood vessel isolation Large blood vessels were isolated as previous described with minor modifications [22] , [60] , [61] . Briefly, brains from Ctr and Nγ1-KO mice were collected, homogenized and centrifuged in dextran solution as described above. Blood vessel pellet was then filtered through 100-μm cell strainers. Large blood vessels trapped by the strainer were collected and homogenized in tissue lysis buffer (100 mM Tris, pH 8, 1% SDS, 200 mM NaCl, 5 mM EDTA, 1 × protease inhibitor cocktail and 1 × phosphatase inhibitor cocktail). PCR and qRT–PCR Total RNA was extracted from primary pericytes using Trizol (Invitrogen), according to manufacturer’s instructions. The RNA was further purified by RNeasy Kit (Invitrogen). Equal amount of total RNA was subjected to reverse transcription using the SuperScript III First-Strand Synthesis System (Invitrogen) as instructed. For PCR, the following primers were used: Laminin γ1 : 5′-TGGGCAGAATCTTTCCTTCT-3′, 5′-ACAGAACTGTCCCCCGTATC-3′; Actin : 5′-ACAGCTGAGAGGGAAATCGT-3′, 5′-TGCTAGGAGCCAGAGCAGTA-3′. For qRT–PCR, laminin γ1 and GAPDH ready-to-use gene expression assays (Invitrogen), master-mix (Applied Biosystems) and cNDA were mixed together and the reaction was run in ABI HT7900 Fast Real-Time PCR System. The expression level of laminin γ1 was normalized to housekeeping gene GAPDH . Lentivirus generation Lentiviruses were purchased from GenTarget. Three shRNA sequences against human ITGA2 (1: 5′-AAGGAAGAGTCTACCTGTTTACGAGTAAACAGGTAGACTCTTCCTT-3′; 2: 5′-GGTGACCAGATTGGCTCCTATCGAGATAGGAGCCAATCTGGTCACC-3′; 3: 5′-CTGGAGTGGCTTTCCTGAGAACGAGTTCTCAGGAAAGCCACTCCAG-3′) and one scrambled sequence (5′-GTCTCCACGCGCAGTACATTTCGAGAAATGTACTGCGCGTGGAGAC-3′) were cloned into GenTarget’s lentiviral shRNA expression vector with RFP-puromycin marker. Sequence-verified lentivectors and lentiviral packaging plasmids were co-transfected into lentivirus production cell lines. The packaged lentiviruses were collected from the medium and filtered through 0.45-μm filter. ITGA2 knockdown Pericytes were plated in laminin-111-coated plates. When cells reached 50% confluence, 8 μg ml −1 polybrene and the appropriate amount of lentivirus were added to reach a final MOI of 2 (2 lentiviruses per cell). Medium was replaced 96 h after transduction. Pericyte lysates were collected 7 days after transduction. Striatum dissection Ctr and Nγ1-KO mice were anaesthetized with avertin (0.02 ml per g of body weight) intraperitoneally. After perfusion with saline, brains were collected and placed under a dissection microscope. Cortices and hippocampi were carefully removed, and the striatum was homogenized in tissue lysis buffer. Western blot Total protein concentration from the lysates was determined using the Bio-Rad protein assay kit. Equal amount of protein was loaded and separated in 10% or 12% SDS-PAGE, followed by transfer to PVDF membrane (Millipore). The membranes were then incubated with anti-AQP4 (Millipore, AB3594, 1:500), anti-occludin (Invitrogen, 71-1500, 1:1,000), anti-ZO-1 (Invitrogen, 40-2200, 1:1,000), anti-Claudin-5 (Invitrogen, 34-1600, 1:1,000), anti-PDGFRβ (Cell Signaling, 3169S, 1:500), anti-SMA (Sigma, F3777, 1:1,000), anti-SM22-α (GeneTex, GTX113561, 1:1,000), anti-integrin α2 (Millipore, AB1936, 1:500), anti-myocardin (R&D, MAB4028, 1:500) and anti-actin (Sigma, A5441, 1:2,000) antibodies at 4 °C overnight, followed by incubation with HRP-conjugated secondary antibodies (Jackson ImmunoResearch Lab). The proteins were visualized by SuperSignal West Pico Chemiluminescent Substrate (Pierce). The density of bands was normalized to actin and quantified using NIH ImageJ. Stereotaxic injection Ad-GFP (SignaGen) and Ad-pGFAP-Cre (kindly provided by Dr Arturo Alvaraz-Buylla) were propagated and purified twice by caesium chloride banding, followed by dialysis in phosphate-buffered saline. Plaque-forming units (3 × 10 8 ) of these adenoviruses were used for injection. Wild-type or F/F mice (2–3 months, 25–35 g, both genders) were anaesthetized as described above. After making an incision, a burr hole was drilled at stereotaxic coordinates of –1 mm posterior to bregma and 2.5 mm lateral from midline. Then, adenoviruses were injected into the brain at the depth of 3.5 mm over 5 min. The needle was kept in place for 2 min to prevent reflux. Seven days after injection, the mice were transcardially perfused and the brains were sectioned. BBB permeability assays Twelve hours before the mice were killed, 2% Evans blue in saline was injected into Ctr, Nγ1-KO and Cγ1-KO mice intraperitoneally at the concentration of 10 μl per g of body weight. After perfusion with saline, the brains were collected and sectioned. BBB breakdown was revealed by visualizing Evans blue at 620 nm under the fluorescence microscope. Mouse IgG was co-immunostained with CD31 and visualized at 555 nm. The quantification of IgG leakage was performed as described previously with minor modifications [62] . Briefly, IgG fluorescent intensity at specific brain regions was determined using ImageJ software. The mean fluorescent intensity per pixel was quantified by using at least nine random images from at least three animals. In addition, 100 μl FITC-Dextran (500 kD, 10 mg ml −1 ) was injected into 2–3 month-old Ctr, Nγ1-KO and Cγ1-KO mice intravenously. After perfusion, brain lysates were collected and the leakage of this dye into the brain was examined using a fluorescence plate reader at 488 nm. Immunohistochemistry Brain sections were immunostained with anti-laminin γ1 (Abcam, AB3297, 1:200), anti-laminin-111 (Sigma, L9393, 1:1,000), anti-laminin α2 (Sigma, L0663, 1:200), anti-laminin α4 (R&D system, AF3837, 1:200), anti-AQP4 (Millipore, AB3594, 1:500), anti-occludin (Invitrogen, 71-1500, 1:500), anti-ZO-1 (Invitrogen, 40-2200, 1:500), anti-Claudin-5 (Invitrogen, 34-1600, 1:500), anti-CD31 (BD Pharmingen, 550274, 1:200), anti-PDGFRβ (eBioscience, 14-1402-82, 1:200 and Cell Signaling, 3169S, 1:200), anti-CD13 (BD Pharmingen, 558744, 1:200), anti-Cre recombinase (Novagen, 69050, 1:2,000) or anti-Ki67 (Millipore, AB9260, 1:1,000) antibodies overnight at 4 °C, followed by fluorescent secondary antibodies (Invitrogen) for 1 hour at room temperature. FITC-conjugated SMA (Sigma, F3777, 1:1000) was used to study pericyte differentiation and distinguish capillaries and large vessels, given that SMA is expressed in arterioles and arteries but not capillaries under normal conditions. After mounting, the brain sections were examined and photographed with an Axiovert 200 (Zeiss) microscopy or Leica confocal microscopy. For quantification, at least nine random images (from at least three animals) with GFP or Cre signal at × 200 magnification were taken and the mean fluorescence intensity was analysed. TUNEL assay Cell death was examined using the In Situ Cell Death Detection Kit, TMR red (Roche), according to the manufacturer’s protocol. Briefly, brain sections were fixed in 4% paraformaldehyde and permeabilized on ice, followed by incubation with TUNEL reaction mixture. After washing, the sections were examined by fluorescence microscopy. EM analysis Two-month-old mice (both genders) were anaesthetized and perfused with PBS following by 0.1 M sodium cacodylate buffer containing 2% paraformaldehyde and 2% glutaraldehyde. After perfusion, the striatum was dissected out and fixed overnight. The tissue was post-fixed in 1% osmium tetroxide and 1% K-ferrocyanide. Next, the tissue was en bloc stained with 2% uranyl acetate and embedded in resin. Ultra-thin sections were cut on a Reichert-Jung Ultracut E microtome and post-stained with 2% uranyl acetate and 1% lead citrate. Sections were examined and photographed using JEOL100CXII at 80 kV. Statistics Results are shown as mean±s.d. Student’s t -test, performed by SPSS Statistics or Microsoft Excel, was used to analyse differences between two groups. How to cite this article: Yao, Y. et al. Astrocytic laminin regulates pericyte differentiation and maintains blood brain barrier integrity. Nat. Commun. 5:3413 doi: 10.1038/ncomms4413 (2014).